Phase seeding of a terahertz quantum cascade laser The amplification of spontaneous emission is used to initiate laser action. As the phase of spontaneous emission is random, the phase of the coherent laser emission (the carrier phase) will also be random each time laser action begins. This prevents phase-resolved detection of the laser field. Here, we demonstrate how the carrier phase can be fixed in a semiconductor laser: a quantum cascade laser (QCL). This is performed by injection seeding a QCL with coherent terahertz pulses, which forces laser action to start on a fixed phase. This permits the emitted laser field to be synchronously sampled with a femtosecond laser beam, and measured in the time domain. We observe the phase-resolved buildup of the laser field, which can give insights into the laser dynamics. In addition, as the electric field oscillations are directly measured in the time domain, QCLs can now be used as sources for time-domain spectroscopy. Controlling the carrier-envelope phase of femtosecond (fs) laser pulses by using active feedback techniques [1] has lead to major advances in frequency metrology [2] and attosecond science [3] , [4] . The phase between consecutive electromagnetic pulses is similarly fixed [5] in time-domain spectroscopy (TDS) [6] . This enables the detection of the electric field in the time domain. As a result, TDS is a powerful technique that allows the dynamics of the complex dielectric response of materials [7] and coherent processes [8] to be investigated as a function of time. In the terahertz (THz) frequency regime, TDS is a widely used technique for THz imaging [9] , biological investigations [10] , non-destructive testing [11] and chemical recognition [12] . THz TDS is implemented by generating THz pulses with a fs laser beam, and synchronously sampling the resulting THz pulses with the same fs laser beam, using techniques such as free-space electro-optic sampling [13] . Time-domain detection of the electric field is made possible, since the phase between successive THz pulses is fixed, even if the carrier-envelope phase of the fs laser pulses is not fixed [5] . This allows multiple-shot averaging of the sampled electric field value. By varying the time delay between the sampling beam and the THz pulse, the field can be characterized as a function of time. However, time-domain detection of free-running sources, such as quantum cascade lasers (QCL) [14] , [15] , cannot be performed with an fs sampling beam. Even with an infinite coherence time, the QCL frequency would need to be an integer multiple of the fs sampling rate (the repetition rate of the fs laser). Otherwise, the carrier phase would vary for each fs sampling pulse, and the resulting multiple-shot average of the sampled electric field value would be zero. Thus, the field of a free-running QCL cannot be measured as a function of time and cannot be used as a source for TDS. This is unfortunate, as many emerging THz applications [16] , [17] take advantage of the small size and high output power [18] of this semiconductor laser. In this article, we show how the carrier phase of the QCL laser emission can be set by coherently injection seeding [19] the QCL with THz pulses having a fixed phase. Here, the seeded field replaces the spontaneous emission of the QCL and sets the carrier phase by triggering the laser emission. Consequently, this enables the electric field of the laser emission to be measured as a function of time over several nanoseconds, from initiation of lasing to the steady-state lasing regime. In contrast to other techniques [2] , [17] , [19] no active feedback or laser stabilization mechanism is necessary for phase-controlled emission. 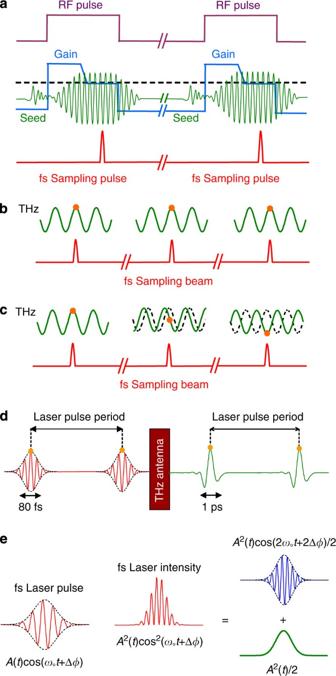Figure 1: Coherent injection seeding of a QCL. (a) A THz pulse injected into the QCL before the gain is turned on initiates lasing. The carrier phase of the QCL emission is then set by the injected THz pulse. (The dashed line represents the value of the gain at laser threshold.) (b) The carrier phase of the emission from a QCL is synchronized with respect to a femtosecond (fs) sampling beam. (c) The carrier phase of the emission from a free-running QCL is not synchronized with respect to a femtosecond sampling beam. The femtosecond sampling beam will measure an average electric field of zero. (d) The phase of the THz pulses is fixed from pulse to pulse even if the carrier phase of the femtosecond laser pulses varies. (e) THz pulses are generated in response to the envelope function (green) of the intensity of the femtosecond laser pulse, which does not depend on the carrier phase . Only the second harmonic response (blue) of the instantaneous intensity depends on the carrier phase Δφ. However, it has no role in the generation of terahertz radiation. To initiate lasing, coherent THz pulses are injected into the QCL when the gain is below threshold, as depicted in Figure 1a . A short time later, the QCL gain is increased above threshold by applying a voltage pulse (radiofrequency (RF) pulse) to the QCL. As no laser field is initially present in the QCL cavity, the gain is unclamped and large amplification can occur [20] . Both the THz pulse and the spontaneous emission in the cavity will be amplified until the intracavity field is large enough to saturate the gain. This clamps the gain to the total losses and results in steady-state lasing. If the field of the injected THz pulses is greater than the spontaneous emission, lasing will be initiated by the THz pulses. The THz pulses will then seed the lasing, as shown in Figure 1a . The carrier phase of the QCL is therefore set by the phase of the coherent THz pulses. This enables the field of the QCL to be measured in the time domain, as shown in Figure 1b . If no injected THz pulse is present, for each RF pulse, the phase of the spontaneous emission (which is random) determines the carrier phase of the QCL, and time-domain detection of the laser emission is not possible, as shown in Figure 1c . It should be noted that, even if the carrier phase of the fs laser pulses varies from pulse to pulse, the phase of the generated THz pulses does not vary ( Fig. 1d ). This is because the THz pulses are created in response to the rectified component of the instantaneous fs laser intensity, which does not depend on the carrier phase of the fs laser ( Fig. 1e ). Figure 1: Coherent injection seeding of a QCL. ( a ) A THz pulse injected into the QCL before the gain is turned on initiates lasing. The carrier phase of the QCL emission is then set by the injected THz pulse. (The dashed line represents the value of the gain at laser threshold.) ( b ) The carrier phase of the emission from a QCL is synchronized with respect to a femtosecond (fs) sampling beam. ( c ) The carrier phase of the emission from a free-running QCL is not synchronized with respect to a femtosecond sampling beam. The femtosecond sampling beam will measure an average electric field of zero. ( d ) The phase of the THz pulses is fixed from pulse to pulse even if the carrier phase of the femtosecond laser pulses varies. ( e ) THz pulses are generated in response to the envelope function (green) of the intensity of the femtosecond laser pulse, which does not depend on the carrier phase . Only the second harmonic response (blue) of the instantaneous intensity depends on the carrier phase Δφ. However, it has no role in the generation of terahertz radiation. Full size image Experimental setup The RF pulses are created by illuminating a fast photodiode with a portion of the fs laser beam. This ensures that the RF pulses are synchronized with the 76 MHz pulse train of the fs laser. The RF pulses are amplified, and a quasi-direct current (DC) offset is then added to the amplified RF pulses with a bias tee. The length of the coaxial cable (which carries the RF pulses) was precisely adjusted so that the edge of the RF pulses arrived at the same time as the injected THz pulses. 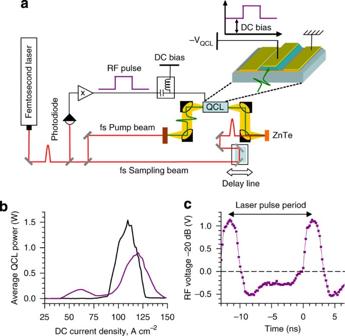Figure 2: Experimental setup. (a) Schematic of the experimental setup. RF voltage pulses are generated from a fast photodiode illuminated by the femtosecond (fs) laser beam (with a centre wavelength of 820 nm). The RF pulses are amplified by a power RF amplifier. A bias tee adds a DC offset to the RF pulses. THz pulses are generated by illuminating a biased interdigitiated antenna with a femtosecond pump beam. The THz pulses are coupled into a facet of the quantum cascade laser (QCL) with parabolic mirrors. The QCL output field from the other facet is measured using electro-optic sampling in a ZnTe crystal with a femtosecond sampling beam. (b) Time-averaged light-current density (L-J) curve of the QCL with RF OFF (black) and RF ON (purple). The QCL output power is measured with a slow pyroelectric detector that averages out any power variations caused by the RF pulses. (c) Instantaneous voltage of RF pulses, measured with a 1 GHz oscilloscope and 20 dB attenuation. The two peaks correspond to two consecutive laser pulses. The negative voltages between RF pulses arise because the RF pulses are alternate current (AC) coupled and the time-averaged RF voltage must therefore be zero. Figure 2a shows a schematic of the experimental setup. THz pulses are generated by illuminating an interdigitated photoconductive antenna [21] with the fs laser beam. The THz pulses are coupled into a facet of a 2 mm-long bound-to-continuum QCL [22] operating at ~2.1 THz. At the opposite facet, the output from the QCL is collected and focused onto a ZnTe crystal along with the fs sampling beam. The THz field inside the ZnTe crystal is then measured using electro-optic sampling [13] . Figure 2: Experimental setup. ( a ) Schematic of the experimental setup. RF voltage pulses are generated from a fast photodiode illuminated by the femtosecond (fs) laser beam (with a centre wavelength of 820 nm). The RF pulses are amplified by a power RF amplifier. A bias tee adds a DC offset to the RF pulses. THz pulses are generated by illuminating a biased interdigitiated antenna with a femtosecond pump beam. The THz pulses are coupled into a facet of the quantum cascade laser (QCL) with parabolic mirrors. The QCL output field from the other facet is measured using electro-optic sampling in a ZnTe crystal with a femtosecond sampling beam. ( b ) Time-averaged light-current density (L-J) curve of the QCL with RF OFF (black) and RF ON (purple). The QCL output power is measured with a slow pyroelectric detector that averages out any power variations caused by the RF pulses. ( c ) Instantaneous voltage of RF pulses, measured with a 1 GHz oscilloscope and 20 dB attenuation. The two peaks correspond to two consecutive laser pulses. The negative voltages between RF pulses arise because the RF pulses are alternate current (AC) coupled and the time-averaged RF voltage must therefore be zero. Full size image The time-average light-current density (L-J) curves are shown with (purple) and without (black) RF pulses applied to the QCL in Figure 2b . With RF pulses applied to the QCL, a local maximum in the time-average L-J curves appears at low current densities. This corresponds to the RF pulses turning on the QCL, with the DC bias below threshold. Figure 2c shows the instantaneous voltage of a typical RF pulse as a function of time. As the RF pulses are amplified by an alternate current (AC) amplifier with a bandwidth of 30 MHz to 1.2 GHz, the time-averaged voltage must be zero. This can be seen in Figure 2c , in which the RF voltage is negative between RF pulses. The negative RF voltage between pulses causes the global maximum of the time-average L-J curve to shift to higher DC current densities in Figure 2b when the RF pulses are on. When a THz pulse is coupled into the input facet of the QCL, it makes a single pass through the QCL. At the output facet, part of the THz pulse is reflected back into the cavity of the QCL, and the other part is transmitted out of the QCL. A portion of the reflected THz pulse will make another round-trip through the cavity and return to the output facet. This process is repeated many times, and the output from the QCL consists of multiple THz pulses separated by the round-trip time of the laser cavity. 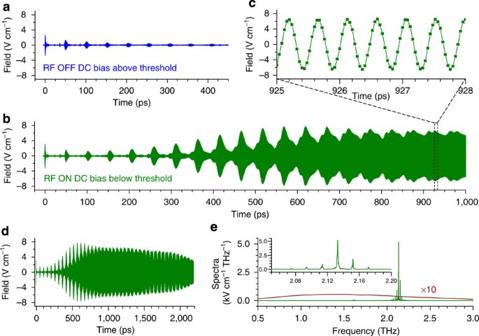Figure 3: Measured fields emitted from the QCL with and without RF pulses. (a) THz pulses transmitted through the QCL, with the RF pulses OFF and the DC bias (93 A cm−2) above threshold. (b) THz pulses transmitted through the QCL, with the RF pulses ON and the DC bias (60 A cm−2) below threshold. (c) Closeup of electro-optically measured field in partbfrom 925 to 928 ps. (d) The electro-optically measured QCL field for the entire scan of 2,200 ps. (e) Spectral amplitude of the electro-optically measured QCL field (green curve) and the antenna output with the QCL removed from the setup (dark red curve). The antenna spectrum is multiplied by a factor of 10 for visual clarity. The inset shows a closeup of the spectral amplitude of the electro-optically measured QCL field. QCL output with the RF pulses OFF Figure 3a (blue curve) shows the transmitted THz pulses with the RF pulses OFF and the QCL biased above the lasing threshold. The THz pulses become elongated and their amplitude becomes smaller as they undergo more and more passes through the QCL. This is similar to previous studies in which THz probe pulses are used to measure the spectral gain of QCLs [23] , [24] , [25] , [26] . In these studies, TDS can only measure the amplification of the injected THz probe pulses. The emission of the QCL cannot be detected, as the carrier phase of the QCL is not locked to the fs sampling rate (the repetition rate of the fs laser). This is clearly evident in Figure 3a ; no sinusoidal steady-state laser field can be measured even though the QCL is biased above threshold and lasing. Figure 3: Measured fields emitted from the QCL with and without RF pulses. ( a ) THz pulses transmitted through the QCL, with the RF pulses OFF and the DC bias (93 A cm −2 ) above threshold. ( b ) THz pulses transmitted through the QCL, with the RF pulses ON and the DC bias (60 A cm −2 ) below threshold. ( c ) Closeup of electro-optically measured field in part b from 925 to 928 ps. ( d ) The electro-optically measured QCL field for the entire scan of 2,200 ps. ( e ) Spectral amplitude of the electro-optically measured QCL field (green curve) and the antenna output with the QCL removed from the setup (dark red curve). The antenna spectrum is multiplied by a factor of 10 for visual clarity. The inset shows a closeup of the spectral amplitude of the electro-optically measured QCL field. Full size image QCL output with the RF pulses ON In strong contrast to the data in Figure 3a , when the DC bias of the QCL is below threshold, but the RF pulses are ON, the amplitude of successive THz pulses in Figure 3b (green curve) significantly increases. The THz pulses increase in amplitude for ~400 ps (from 200 to 600 ps), which is on the order of the rise time of the RF pulses. For much longer time periods, successive THz pulses merge together, and the field becomes quasi-monochromatic, as shown in Figure 3c . At these time scales, the THz field in the QCL cavity has saturated the gain (clamped it to the total losses), and the injected THz seed pulse has become the laser field of the QCL. The field amplitude emitted by the QCL (in the absence of injected THz pulses) is calculated from power measurements to be 8.1 V cm −1 . This is in good agreement with the measured amplitude (6.4 V cm −1 ) in Figure 3c , considering that the frequency response of the ZnTe crystal is not taken into account. A small secondary THz pulse, caused by reflections in the substrate of the THz-generating antenna, can be observed at ~35 ps in Figure 3a . The secondary THz pulse is also amplified by the unclamped gain and alters the shape of the field envelope as the field in the QCL builds up. Interference from the secondary seed pulse also contributes to the ripples of the field envelope at much longer time periods (>800 ps) in Figure 3b . In Figure 3d , the field is shown for the entire scan of 2,200 ps. After the initial rise of the THz pulses, a slight decrease of the peak field is observed after 600 ps. This could be due to a small overshoot of the THz field with respect to the steady-state lasing value, or to a voltage deviation of the RF pulse from an ideal rectangular pulse shape (as shown in Fig. 2c ). After a slight decrease of the peak amplitude (that takes place after 600 ps), the peak amplitude is approximately flat until ~2,000 ps, at which time the RF pulse begins to turn OFF. In Figure 3e , the spectral amplitude of the field in Figure 3d is compared with the spectral amplitude of an input THz pulse produced by the THz-generating antenna, with the QCL removed from the setup. The spectral amplitude of the QCL field (measured by electro-optic sampling) is two orders of magnitude larger than that of the antenna at 2.13 THz. In the inset of Figure 3e , it can be seen that the measured QCL field consists of a main line at 2.13 THz surrounded by several smaller lines with a spacing of ~20 GHz, which corresponds to the round-trip time (~50 ps) of the laser cavity. Saturation measurements To further confirm that injection seeding is taking place, saturation measurements are performed on the QCL by varying the amplitude of the input THz pulses. To change the amplitude of the THz pulses, we varied the voltage applied to the THz-generating antenna. The amplitude of the THz pulses was confirmed to be proportional to the voltage applied to the antenna (see Supplementary Figure S1 ). 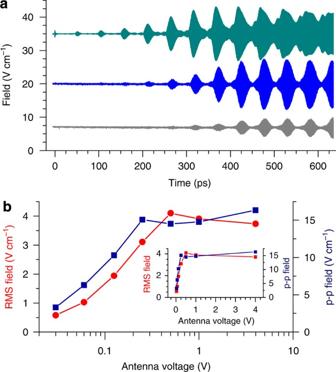Figure 4: Seed pulse saturation measurements. (a) Electro-optically measured fields of the QCL output for various input THz pulse amplitudes. The THz pulse amplitude is varied by changing the antenna voltage. (The THz pulse amplitude is proportional to the antenna voltage.) Output fields are shown for input THz pulses generated with an antenna bias of 1 V (green curve), 0.25 V (blue curve) and 0.06 V (grey curve). The QCL DC bias (66 A cm−2) is below threshold. (b) The peak-to-peak (p-p) amplitude and root mean square (RMS) of the THz fields in partafor time periods >500 ps versus the antenna voltage (logarithmic scale). Inset—partb, on a linear voltage scale. For the data in Figure 3 , the antenna voltage was 4 V. Figure 4a shows output fields of the QCL for different amplitudes of the input THz pulses. For each field in Figure 4a , the antenna voltage, and hence the input THz amplitude, varies by a factor of 4. It is particularly striking that for time periods >500 ps (after the intracavity field buildup time), the output amplitude hardly changes for antenna voltages of 0.25 and 1 V, even though the input THz pulse amplitude differs by a factor of 4. The root mean square and peak-to-peak (p-p) amplitude of the fields from 500 to 640 ps are plotted in Figure 4b as a function of the antenna voltage. The kink in Figure 4b at 0.25 V shows a clear saturation of the output field. This implies that the QCL gain is clamped (that is, saturated) by the amplified THz input pulses, and the THz input pulses initiate (that is, seed) laser action for antenna voltages >0.25 V. For antenna voltages <0.25 V, the measured QCL output field depends on the input THz pulse amplitude. This implies that the QCL gain is then clamped by the intracavity amplified spontaneous emission, rather than by the injected THz pulses. As the amplified spontaneous emission has a carrier phase that varies randomly for each fs sampling pulse, its field cannot be detected with the fs sampling beam. Figure 4: Seed pulse saturation measurements. ( a ) Electro-optically measured fields of the QCL output for various input THz pulse amplitudes. The THz pulse amplitude is varied by changing the antenna voltage. (The THz pulse amplitude is proportional to the antenna voltage.) Output fields are shown for input THz pulses generated with an antenna bias of 1 V (green curve), 0.25 V (blue curve) and 0.06 V (grey curve). The QCL DC bias (66 A cm −2 ) is below threshold. ( b ) The peak-to-peak (p-p) amplitude and root mean square (RMS) of the THz fields in part a for time periods >500 ps versus the antenna voltage (logarithmic scale). Inset—part b , on a linear voltage scale. Full size image Seed amplification A laser can be considered as the ultimate amplifier: when initially turned on, it takes a very small signal (the spontaneous emission), and amplifies it to the steady-state laser value. Injection seeding can be simply thought of as amplification of an input seed to the value of the laser field. We calculate the amplification factor using the QCL field from one round-trip time as the output, and the THz field from the antenna (with the QCL removed from the setup) as the input. 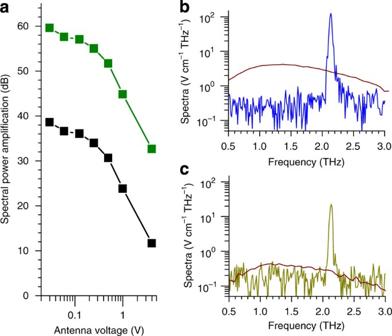Figure 5: Amplification of the seed pulse. (a) Power spectral amplification factors for the fields inFigure 4(from 557 to 608 ps; one round-trip time interval) versus antenna voltage. Green—including input coupling losses. Black—excluding input coupling losses. The THz pulse amplitude is proportional to the antenna voltage. (b) Antenna voltage 0.25 V. Blue curve—spectra of the QCL output from 557 to 608 ps. Dark red curve—spectra of the antenna output with the QCL removed from the setup. (c) Antenna voltage 0.03 V. Dark yellow curve—spectra of the QCL output from 557 to 608 ps. Dark red curve—spectra of the antenna output with the QCL removed from the setup. The power amplification factor is shown in Figure 5a with and without taking account of the large coupling losses into the QCL facet. The largest amplification factor occurs for THz input pulses generated with antenna voltages <0.25 V. These THz pulses are in the linear amplification regime of Figure 5a and do not saturate the QCL gain. As a consequence, the amplification factor is relatively flat in Figure 5a for antenna voltages <0.25 V. In contrast for THz input pulses with antenna voltages >0.25 V, the amplification factor decreases as the THz pulse amplitude increases, as these THz pulses saturate the QCL output. The QCL output spectra from one round-trip time interval (557–608 ps) and the THz input pulse spectra are shown in Figure 5b and c for antenna voltages of 0.25 and 0.03 V. Unlike Figure 3e , the QCL output spectra in Figure 5b and c both consist of a single peak. The spectral lines in Figure 3e are the result of multiple reflections from the laser cavity facets and are only present for time durations greater than the round-trip time. Figure 5: Amplification of the seed pulse. ( a ) Power spectral amplification factors for the fields in Figure 4 (from 557 to 608 ps; one round-trip time interval) versus antenna voltage. Green—including input coupling losses. Black—excluding input coupling losses. The THz pulse amplitude is proportional to the antenna voltage. ( b ) Antenna voltage 0.25 V. Blue curve—spectra of the QCL output from 557 to 608 ps. Dark red curve—spectra of the antenna output with the QCL removed from the setup. ( c ) Antenna voltage 0.03 V. Dark yellow curve—spectra of the QCL output from 557 to 608 ps. Dark red curve—spectra of the antenna output with the QCL removed from the setup. Full size image In the measurements presented above, the QCL is seeded by an external THz pulse from a photoconductive antenna. The latter can be easily eliminated by directly generating the THz pulse on the QCL by exciting the facet with a fs laser pulse [27] . As well as simplifying the TDS setup, this would avoid the large coupling losses associated with injecting free-space THz radiation into QCL waveguides, as the THz pulse would be automatically coupled into the QCL cavity. Furthermore, the technique of coherent injection seeding is not limited to the far infrared. It should also be possible to phase-seed mid-infrared QCLs and detect their phase-resolved output in the time domain. Indeed, investigations of the gain of mid-infrared QCLs using TDS have already begun [26] , [28] . Besides using the QCL as an active device, the phase-resolved dynamics of the QCL field can also be explored. This could enable the investigation of mode-locked behaviour in QCLs. [29] , [30] The dynamics of the buildup of the laser field can also be investigated from the initiation of lasing to the steady state. It is interesting to consider the results in the context of the frequency domain. For very long time scales, the output of the injection-seeded QCL consists of a train of THz pulses (with nanosecond durations) emitted at the fs laser repetition rate (~13 ns). The spectrum of this QCL pulse train should mathematically consist of several spectral lines ( f QCL ), such that f QCL = mf rep + f o , where m is an integer, f rep is the fs laser repetition frequency and f o is an offset frequency [1] . If the carrier phase is constant and does not vary between pulses, the frequency offset ( f o ) will be exactly equal to zero. [1] This enables synchronized fs sampling of the QCL emission, and time-resolved detection of the QCL field. In contrast, for non-synchronized fs sampling [31] and other phase-locked QCLs [32] , f o is not zero, which inhibits time-resolved detection of the field. In conclusion, the carrier phase of a QCL can be set by coherent injection seeding without any active feedback or laser stabilization techniques. This enables the phase-resolved laser emission to be measured in the time domain and the QCL to be used as a powerful source for TDS. Description of the QCL The QCL device was a 2 mm-long and 250 μm-wide QCL that lased at ~2.1 THz. A plasmon waveguide was used for mode confinement. The active region of the device consisted of alternatively spaced layers of GaAs and Al 10 Ga 90 As , with thicknesses of 5 /126/ 44 /120/ 32 /124/ 30 /132/ 24 /144/ 10 /118/ 10 /144 nm. The device was bounded to a Cu heat sink bar with indium and attached to a cold finger of a helium flow cryostat that was cooled to 4.5 K. THz pulse generation and detection THz pulses were generated by illuminating an interdigitated photoconductive antenna on GaAs with an fs laser (~1 W average power, ~80 fs pulse duration, 76 MHz). The antenna had a finger spacing of 1.5 μm and a period of 6 μm. The macroscopic active area of the antenna was a 500 μm circle. The 500 μm-thick GaAs substrate was attached to a 1 mm high-resistivity Si wafer to extend the echo time between multiple reflections in the substrate. The generated THz pulses were collected by a f #2 parabolic mirror and focused onto a QCL facet with a f #1.67 parabolic mirror. The windows of the cryostat were thin quartz windows, unlike the tsurupica windows used in previous studies. After exiting the QCL through the opposite facet, the THz pulses were collimated with a f #2 parabolic mirror and refocused with a f #1 parabolic mirror onto a 200 μm-thick <110> ZnTe crystal. The ZnTe crystal was mounted on a 2 mm-thick <100> ZnTe crystal. (The <100> crystal has a null electro-optic effect in this geometry.) This extended the time between echoes in the ZnTe. The THz electric field in the 200 μm ZnTe crystal was then measured with an fs sampling beam using electro-optic sampling. Generation and amplification of RF voltage pulses locked to the fs laser repetition rate RF voltage pulses were created by illuminating a fast Si photodiode with a portion of the fs laser beam. The RF pulses were sent into a preamplifier that was used as a limiting amplifier to convert the RF pulses to square-like pulses with a relatively flat top. A 50-Ω switch enabled the RF pulse train to be gated at kHz frequencies. A variable voltage-controlled attenuator was used to vary the amplitude of the RF pulses, which were then sent into an RF power amplifier (30–1,200 MHz). Fixed coaxial attenuators were used throughout the RF setup to control the RF power level. The amplified RF pulses were then combined with a DC bias (modulated at 10 kHz) in a bias tee. The DC bias was modulated at 10 kHz to enable detection with a lock-in amplifier. The same 10 kHz modulation was also applied to the RF pulses with the 50-Ω switch. The combined RF pulses and the quasi-DC offset were applied to the QCL sample. The leads connecting the sample to the coaxial cable were made as short as possible to avoid RF reflections. The RF input pulses and reflected RF output pulses could be monitored by using a two port 20-dB directional coupler (40–1,000 MHz). The RF pulses split off by the directional coupler were measured with a 1 GHz oscilloscope across a 50 Ω load. Adjusting the arrival time of the RF electrical pulses To ensure that the arrival of the RF pulses coincided with the arrival of the THz pulses into the QCL cavity, the length of the coaxial cable in the RF setup was adjusted. Fine-length adjustment could be made by adding and subtracting several Sub miniature version A (SMA) male–female adapters. Because of the amount of RF components and the geometry of the experimental setup, the path length for the RF pulses was much longer than the path length for the fs and THz pulses. Because of this, a single fs laser pulse could not be used to trigger the same THz pulse and RF pulse. Instead the THz pulses were triggered two laser pulses (~26 ns) after the RF electrical pulses were triggered. Modulation and data-taking scheme for lock-in detection The antenna was modulated at 20 kHz with a 50% duty cycle and the QCL and 50 Ω switch bias pulses were modulated at 10 kHz with a 25% duty cycle. The individual QCL bias pulses and the antenna bias pulses had the same time duration, and were synchronized in time. There were twice as many antenna bias pulses as QCL bias pulses, and for every other antenna bias pulse, the QCL bias pulse was alternatively ON and then OFF. The 10 kHz modulation was used as the reference for the lock-in amplifier. Because of the synchronized bias pulse scheme, the lock-in amplifier detected the difference between the THz field with the QCL and RF ON, and the THz field with the QCL and RF OFF ( E ( t ) QCL, RF ON − E ( t ) QCL, RF OFF ). However, this distinction is only important for a single pass through the QCL. For multiple passes, the loss within the QCL is so great that E ( t ) QCL,RF OFF is essentially zero, and the measured field is for all practical purposes E ( t ) QCL, RF ON . Steady-state value determination for the field emitted by the QCL We can determine whether the QCL field (measured by electro-optic detection in Figure 3c ) is comparable with the field emitted by the QCL in the steady-state regime (with no THz pulses injected into the laser). To do this, we measure the c.w. power of the THz pulse generated by the antenna ( P Ant ) with the QCL removed from the setup, and the c.w. power of the QCL emission ( P QCL ) (with no seeding THz pulses) under identical conditions with a pyroelectric detector. If we assume that the spot size of the QCL emission and the THz pulses are identical in the ZnTe crystal, then where E Ant ( t ) is the field of the THz pulse from the antenna (with the QCL removed), E QCL ( t ) is the field of the c.w. QCL emission and T is the period of the fs laser pulse (~13 ns). By measuring E Ant ( t ) using electro-optic sampling, the root mean square of the THz pulse can be determined, and the amplitude of the c.w. QCL emission can be calculated. Note that, besides implicitly assuming identical spot sizes in the ZnTe crystal, equation (1) also neglects the frequency response of the ZnTe and pryoelectric detectors. We find an amplitude of 8.1 V cm −1 for the steady-state QCL field, which is in good agreement with the time-resolved electro-optically measured field of 6.4 V cm −1 in Figure 3c . How to cite this article: Oustinov, D. et al . Phase seeding of a terahertz quantum cascade laser. Nat. Commun. 1:69 doi: 10.1038/ncomms1068 (2010).